Pharmacological targeting of the mammalian clock regulates sleep architecture and emotional behaviour Synthetic drug-like molecules that directly modulate the activity of key clock proteins offer the potential to directly modulate the endogenous circadian rhythm and treat diseases associated with clock dysfunction. Here we demonstrate that synthetic ligands targeting a key component of the mammalian clock, the nuclear receptors REV-ERBα and β, regulate sleep architecture and emotional behaviour in mice. REV-ERB agonists induce wakefulness and reduce REM and slow-wave sleep. Interestingly, REV-ERB agonists also reduce anxiety-like behaviour. These data are consistent with increased anxiety-like behaviour of REV-ERBβ-null mice, in which REV-ERB agonists have no effect. These results indicate that pharmacological targeting of REV-ERB may lead to the development of novel therapeutics to treat sleep disorders and anxiety. Circadian rhythms play an essential role in aspects of physiology and behaviour including the sleep–wake cycle, body temperature, blood pressure and renal function. At the molecular level, these circadian rhythms oscillate as a function of a feedback loop in gene expression where heterodimers of BMAL1 and CLOCK (or NPAS2 ) (the positive limb) activate the expression of the Cryptochrome ( CRY ) and Period ( PER ) genes (the negative limb). Once CRY and PER have reached a critical level of expression, they are able to block the stimulatory effect of the CLOCK/BMAL1 complex on their own promoters, completing the loop. The nuclear receptors REV-ERBα and REV-ERBβ play an important role in regulation of the molecular clock where they directly suppress the expression of genes of the positive limb of the clock including CLOCK , BMAL1 and NPAS2 (refs 1 , 2 , 3 ). Rev-erb α /Rev-erbβ- deficient mice display profound alterations in circadian behaviour as well as expression of clock genes [4] . Normal oscillations in metabolic function are regulated by the circadian clock, and disruption in the normal function of the clock leads to metabolic disorders including diabetes, obesity and atherosclerosis [5] , [6] , [7] , [8] . We recently demonstrated that synthetic REV-ERB agonists altered both central and peripheral clock gene expression, as well as modulated the metabolic state in vivo [9] , [10] . Pharmacological activation of REV-ERB led to increased energy expenditure, loss of fat mass and improved plasma lipid profiles in mice [9] . We also observed increased oxidative capacity in skeletal muscle in mice that was associated with increased exercise endurance after treatment with a REV-ERB agonist [11] . Thus, direct targeting of a molecular clock component can alter the metabolic state and improve metabolic function. Dysregulation of the circadian rhythm is associated with many disorders including metabolic diseases and neuropsychiatric disorders including bipolar disorder, anxiety, depression, schizophrenia and sleep disorders [12] , [13] , [14] , [15] . In this report, we examined the effects of REV-ERB agonists on patterns of sleep and wakefulness, and found that the compounds increase wakefulness. Furthermore, during this analysis we found that the compounds also decreased anxiety-like behaviour. Thus, we hypothesize that targeting components of the mammalian clock with small molecules may provide therapeutics for treatment of sleep disorders and anxiety disorders. Regulation of sleep by synthetic REV-ERB agonists The ‘master’ circadian clock located in the suprachiasmatic nucleus of the hypothalamus plays an essential role in regulation of sleep [16] and given this close relationship, we sought to investigate the effect of pharmacological activation of REV-ERB on patterns of sleep and wakefulness. Although we observed alterations in circadian wheel running activity previously [9] , the effect on sleep was not clear. To investigate this, we administered a REV-ERB agonist, SR9011, to mice and examined the effect on sleep and wakefulness by electroencephalogram (EEG). As illustrated in Fig. 1a , mice displayed a normal nocturnal profile with low wakefulness and high, slow-wave sleep (SWS) and paradoxical sleep—rapid eye movement (REM) sleep during the daytime (zeitgeiber time 0 (ZT0) to ZT12). Mice were administered SR9011 (100 mg kg −1 , intraperitoneally (i.p.)) or vehicle at ZT6 when Rev-erb expression is at its peak [9] . SR9011-treated mice displayed a large increase in wakefulness that was maintained for 2 h post injection ( Fig. 1a , top panel). As expected, this corresponded to a decrease in SWS and REM sleep during the same time period ( Fig. 1a , bottom panels). Latency to enter SWS and REM sleep after administration of SR9011 was increased as illustrated in Fig. 1b . At the onset of the dark period (ZT12), vehicle-treated mice displayed a normal, rapid increase in wakefulness (and decrease in SWS and REM sleep), while this effect was delayed in SR9011-treated mice ( Fig. 1a ). A normal pattern of sleep was observed after this recovery period ~12 h after the initial injection. Analysis of sleep architecture after the single injection of SR9011 at ZT6 revealed effects on both SWS and REM sleep architecture ( Fig. 2 ). Following injection of SR9011, the number of episodes of SWS increased while their duration was shortened ( Fig 2a,b ). 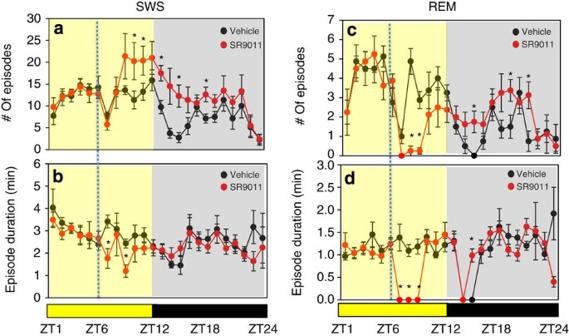Figure 2: Administration of SR9011 alters sleep architecture. Effect of SR9011 administered at ZT6 (analysis of data fromFig. 1a) on SWS (number of episodes (a) and episode duration (b)), and on REM sleep (number of episodes (c) and episode duration (d)). Potential differences between treatments were assessed by repeated-measures two-way ANOVA followed by Bonferronipost hoctest with significance *P<0.05. REM sleep was also affected and was more impressive with REM sleep episodes and duration being nearly completely suppressed for 3 h following administration of SR9011 ( Fig 2c,d ). The sleep recovery period that was observed following transition to dark was also observed in the sleep architecture. Episodes of SWS were increased in SR9011-treated mice from ZT13-15, while SWS duration remained constant ( Fig 2a,b ). Episodes of REM sleep were also elevated after transition to dark with SR9011 treatment ( Fig. 2c ). No effect of SR9011 treatment was observed on EEG power ( Supplementary Fig. 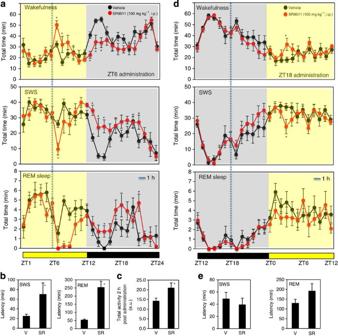1A ). Figure 1: SR9011 induces wakefulness and suppresses sleep. (a) Mice injected with The REV-ERB agonist SR9011 (i.p. 100 mg kg−1) at ZT6 display an increase in wakefulness as detected by EEG. (b) SR9011 increases SWS and REM sleep latency. (c) Locomotor telemetry data indicating an increase in movement during the period 2 h after ZT6 injection of SR9011. (d) Mice injected with SR9011 (i.p. 100 mg kg−1) at ZT18 fail to demonstrate increased wakefulness. (e) SR9011 does not alter SWS and REM sleep latency (ZT18 injection). Data are expressed mean±s.e.m. All EEG graphs are plotted per 1 h for a 24-h period. Values are mean±s.e.m (n=8 for EEG studies (a,b,d,e) andn=6 for telemetry studies (c)). Within the EEG studies (wakefulness, SWS and REM sleep), potential differences between treatments were assessed by repeated measure two-way analysis of variance (ANOVA) followed by Bonferronipost hoctest. In panels examining latency and activity, differences between treatment groups (vehicle versus SR) were assessed by a two-tailed Student’st-test with significance *P<0.05. In all experiments, mice were maintained on a 12 h:12 h L:D cycle. Figure 1: SR9011 induces wakefulness and suppresses sleep. ( a ) Mice injected with The REV-ERB agonist SR9011 (i.p. 100 mg kg −1 ) at ZT6 display an increase in wakefulness as detected by EEG. ( b ) SR9011 increases SWS and REM sleep latency. ( c ) Locomotor telemetry data indicating an increase in movement during the period 2 h after ZT6 injection of SR9011. ( d ) Mice injected with SR9011 (i.p. 100 mg kg −1 ) at ZT18 fail to demonstrate increased wakefulness. ( e ) SR9011 does not alter SWS and REM sleep latency (ZT18 injection). Data are expressed mean±s.e.m. All EEG graphs are plotted per 1 h for a 24-h period. Values are mean±s.e.m ( n =8 for EEG studies ( a , b , d , e ) and n =6 for telemetry studies ( c )). Within the EEG studies (wakefulness, SWS and REM sleep), potential differences between treatments were assessed by repeated measure two-way analysis of variance (ANOVA) followed by Bonferroni post hoc test. In panels examining latency and activity, differences between treatment groups (vehicle versus SR) were assessed by a two-tailed Student’s t -test with significance * P <0.05. In all experiments, mice were maintained on a 12 h:12 h L:D cycle. Full size image Figure 2: Administration of SR9011 alters sleep architecture. Effect of SR9011 administered at ZT6 (analysis of data from Fig. 1a ) on SWS (number of episodes ( a ) and episode duration ( b )), and on REM sleep (number of episodes ( c ) and episode duration ( d )). Potential differences between treatments were assessed by repeated-measures two-way ANOVA followed by Bonferroni post hoc test with significance * P <0.05. Full size image In a separate experiment, we implanted mice with transmitters to detect locomotion by telemetry. Using the same paradigm (12 h:12 h light:dark (L:D) and injection at ZT6), we monitored locomotor activity following injection of SR9011 or vehicle. Mice receiving SR9011 displayed considerably more locomotor activity following injection than vehicle consistent with an increase in wakefulness ( Fig. 1c ). The telemetry units we used also enabled measurement of core temperature and we assessed core temperature under the same paradigm that we assessed sleep–wakefulness patterns. As shown in Supplementary Fig. 2 , we observed the expected circadian pattern of body core temperature with higher temperatures noted during periods of darkness that are associated with wakeful mice. On administration of SR9011 or vehicle at ZT6, we observed an abrupt increase in core temperature, which we attribute to the waking of the animals due to administration that we observed in the EEG as well ( Supplementary Fig. 2A ). Following administration, mice treated with vehicle displayed core temperatures that returned to levels consistent with pre-administration levels; however, core temperatures in the SR9011-treated mice remained elevated relative to vehicle-treated mice for ~2 h ( Supplementary Fig. 2A ). This elevation was ~0.5 °C, which is smaller than the elevation typically observed with wakefulness during the dark period. Interestingly, there was no difference in core temperatures of mice treated with vehicle or SR9011 during the dark period where we have clearly observed a sleep recovery period by EEG. This indicates that although the mice are recovering in terms of sleep, the core temperature is elevated to levels equivalent to wakefulness. Next, we examined the effect of a REV-ERB agonist on sleep patterns when administered during the animals’ wakeful period. SR9011 or vehicle was administered to mice at ZT18, a time when the percentage of mice in a wakeful state is very high. We observed no distinction in sleep–wakefulness patterns between SR9011 and vehicle treatment; furthermore, beginning at ZT0 the mice entered their sleep phase normally ( Fig. 1d ). Latency to enter SWS and REM sleep was unaffected when the REV-ERB agonist was administered at ZT18 ( Fig. 1e ). Thus, our data indicate that pharmacological activation of REV-ERB leads to increased wakefulness, but this effect is dependent on the time of day the compound is administered. To further assess the specificity of this effect for REV-ERB agonists, we examined the effects of a distinct synthetic REV-ERB agonist, SR9009, on sleep architecture under L:D conditions. As shown in Fig. 3a , the effect of SR9009 was very similar to SR9011 with induction of wakefulness and suppression of SWS and REM sleep followed by a recovery period during the subsequent dark period. Latency to enter SWS and REM sleep was also extended following SR9009 injection ( Fig. 3b ). Similar to SR9011-treated mice, mice treated with SR9009 returned to normal patterns of wakefulness/sleep 12 h after administration. Assessment of sleep architecture revealed a similar profile to that observed with administration of SR9011. After administration of SR9009 at ZT6, there was a general increase in episodes of SWS with a decrease in episode duration ( Fig. 4a,b ). The only distinction between SR9011 and SR9009 is a short delay in the increased SWS episode number where the number of episodes is actually decreased for one time point. REM sleep is also similarly affected with REM sleep episodes and episode duration suppressed following administration of SR9009 ( Fig. 4c,d ). The effect on sleep recovery was also observed after SR9009 treatment where the number of episodes of SWS and REM sleep were elevated after transition to the dark period ( Fig. 4a,c ). No effect on EEG power was observed ( Supplementary Fig. 1B ). 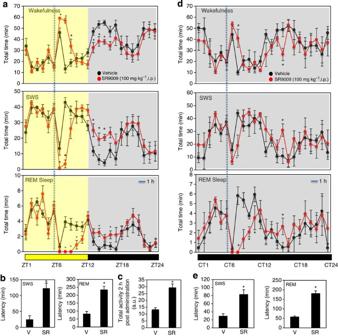Figure 3: SR9009 induces wakefulness and suppresses sleep. (a) Mice injected with the REV-ERB agonist SR9009 (i.p. 100 mg kg−1) at ZT6 display an increase in wakefulness as detected by EEG. (b) SR9009 increases SWS and REM sleep latency. (c) Locomotor telemetry data indicating an increase in movement during the period 2 h after ZT6 injection of SR9011. Mice ina,bandcwere maintained under 12 h:12 h L:D conditions. (d) Mice injected with SR9009 (i.p. 100 mg kg−1) at CT6 under constant dark conditions show increased wakefulness. (e) SR9009 increases SWS and REM sleep latency when injected at CT6 under constant dark conditions. Data are expressed as mean±s.e.m. All EEG graphs are plotted per 1 h for a 24-h period. Values are mean±s.e.m. (n=8 for EEG studies andn=6 for telemetry studies). (c) Within the EEG studies (wakefulness, SWS and REM sleep), potential differences between treatments were assessed by repeated measures two-way ANOVA followed by Bonferronipost hoctest. In panels examining latency and activity, differences between treatment groups (vehicle versus SR) were assessed by a two tailed Student’st-test with significance *P<0.05. Experiments were performed at least twice. Figure 3: SR9009 induces wakefulness and suppresses sleep. ( a ) Mice injected with the REV-ERB agonist SR9009 (i.p. 100 mg kg −1 ) at ZT6 display an increase in wakefulness as detected by EEG. ( b ) SR9009 increases SWS and REM sleep latency. ( c ) Locomotor telemetry data indicating an increase in movement during the period 2 h after ZT6 injection of SR9011. Mice in a , b and c were maintained under 12 h:12 h L:D conditions. ( d ) Mice injected with SR9009 (i.p. 100 mg kg −1 ) at CT6 under constant dark conditions show increased wakefulness. ( e ) SR9009 increases SWS and REM sleep latency when injected at CT6 under constant dark conditions. Data are expressed as mean±s.e.m. All EEG graphs are plotted per 1 h for a 24-h period. Values are mean±s.e.m. ( n =8 for EEG studies and n =6 for telemetry studies). ( c ) Within the EEG studies (wakefulness, SWS and REM sleep), potential differences between treatments were assessed by repeated measures two-way ANOVA followed by Bonferroni post hoc test. In panels examining latency and activity, differences between treatment groups (vehicle versus SR) were assessed by a two tailed Student’s t -test with significance * P <0.05. Experiments were performed at least twice. 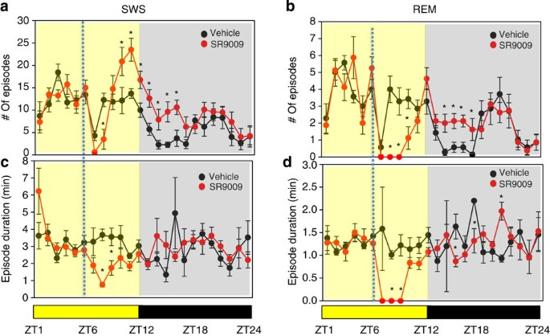Figure 4: Administration of SR9009 alters sleep architecture. Effect of SR9009 administered at ZT6 (analysis of data fromFig. 3a) on SWS (number of episodes (a) and episode duration (b)) and on REM sleep (number of episodes (c) and episode duration (d)). Potential differences between treatments were assessed by repeated measures two-way ANOVA followed by Bonferronipost hoctest with significance *P<0.05. Full size image Figure 4: Administration of SR9009 alters sleep architecture. Effect of SR9009 administered at ZT6 (analysis of data from Fig. 3a ) on SWS (number of episodes ( a ) and episode duration ( b )) and on REM sleep (number of episodes ( c ) and episode duration ( d )). Potential differences between treatments were assessed by repeated measures two-way ANOVA followed by Bonferroni post hoc test with significance * P <0.05. Full size image With this particular experiment, we continued to observe the pattern of sleep–wakefulness for 48 additional hours to determine whether there was any effect on circadian patterns of sleep. As shown in Supplementary Fig. 3 , we did not observe any alterations in the pattern of sleep in response to SR9009 after the first day of administration. Assessment of core body temperature following administration of SR9009 yielded similar results as did SR9011 administration ( Supplementary Fig. 2B ). Immediately following administration of SR9009, core temperature was elevated, but not to levels that are normally associated with wakefulness during darkness. In addition, as observed with SR9011 administration, increased sleep after transition to the dark period was not associated with lower core temperatures ( Supplementary Fig. 2B ). Assessment of locomotion by telemetry in mice injected with SR9011 or vehicle revealed a response that was consistent with increased wakefulness induced by SR9011 treatment ( Fig. 3c ). Previously, we demonstrated that the effects of REV-ERB agonists on wheel-running behaviour were distinct based on whether the mice were maintained on a 12 h:12 h L:D cycle or in complete darkness [9] . We performed an identical experiment to that described in Fig. 3a monitoring EEG, except the animals were maintained in complete darkness, which was initiated 2 days before injection. The effects of SR9009 administration at CT6 under constant darkness were very similar to those obtained under L:D conditions with increased wakefulness and decreased SWS and REM sleep observed ( Fig. 3d ). Increased latency to enter SWS and REM sleep following injection was also observed with SR9009 treatment ( Fig. 3e ). Regulation of anxiety by synthetic REV-ERB agonists Polymorphisms in clock genes ( RORA , CRY1 , RORB , NR1D1 , NPAS2 , CRY2 , PER2 , PER3 and BMAL1 ) have been linked to bipolar, depressive and anxiety disorders in human [17] , [18] , [19] , [20] , [21] , [22] , [23] , [24] . Thus, the ability to modulate the patterns of expression of the clock genes by the REV-ERB agonists may provide a mechanism to influence these disorders. Mice with a disrupted Clock gene display a behavioural profile similar to human mania that included hyperactivity, decreased sleep, lowered anxiety and an increase in reward value for cocaine [25] . A second group established that the Clock mutant mice exhibited increased exploratory activity and escape seeking behaviour consistent with lower levels of anxiety [26] . The positive limb of the circadian clock is under direct positive transcriptional control by the retinoic acid receptor-like orphan receptors [27] , and consistent with loss of Clock gene expression associated with reduced anxiety-like behaviour, mice harbouring a null mutation in the Rorβ gene also are less prone to display anxiety-like behaviour [28] . These data suggest that targeting components of the molecular clock may be an effective method to influence anxiety behaviour. More specifically, based on the genetic data described above, suppression of the positive limb of the clock, such as by activation of REV-ERB activity, may suppress anxiety. In previous experiments with S9011 and SR9009, where we examined the effects of REV-ERB agonism on metabolic rate [9] (chronic twice per day dosing (b.i.d.) (ZT0 and ZT12)), we noted alterations in behaviour that suggested alterations in anxiety-like behaviour. Based on the links between the circadian rhythm and anxiety discussed above, as well as our preliminary observations, we examined the effects of REV-ERB agonists on anxious behaviour more closely. Mice were administered SR9011 chronically as was performed for previous assessments of effects on metabolic parameters (3–10 days; 100 mg kg −1 , b.i.d., i.p. ; details provided in the Methods as illustrated in Supplementary Fig. 4 ) before beginning an open-field assay to assess anxiety-like behaviour. In an open-field assay, mice treated with SR9011 spent considerably more time in the centre of the field, but displayed no change in total distance travelled ( Fig. 5a,b ). This anxiolytic effect was confirmed in several other behavioural assays. Consistent with the anxiolytic activity of SR9011, mice treated with the drug spent considerably more time in the open arms in an elevated plus maze (EPM) assessment ( Fig. 5c ). In addition, the mice displayed a greater number of open-arm entries ( Fig. 5d ). We also assessed the effect of SR9011 on neophobia exhibited by mice in a novel object assay. Mice treated with SR9011 spent 6.5-fold more time near the novel object consistent with anxiolytic activity ( Fig. 5e,f ). Anxiolytic activity was also assessed in a light–dark box assay and as shown in Fig. 5g . Mice administered SR9011 spent considerably more time in the light portion of the box, again consistent with anxiolytic activity of the REV-ERB agonist. Mice displayed no change in the number of transitions between the two boxes in this assay ( Fig. 5h ). In a social interaction assay (SIA) mice treated with SR9011 displayed increased interaction with a novel mouse relative to vehicle-treated animals ( Fig. 5i ). Finally, we assessed the effect of the drug in the marble-burying assay, where mice are introduced into cages with marbles on the surface of the bedding. Mice will naturally bury the marbles to remove the stressful stimuli and effects of anxiolytics can be readily assessed by reduced marble-burying activity. As demonstrated in Fig. 5j , mice administered SR9011 buried only 50% of the marbles that mice administered vehicle did. This anxiolytic effect was dose dependent ( Fig. 5k ) and the potency (ED 50 =61 mg kg −1 ) compares favourably with the potency of SR9011 effects on circadian rhythm (ED 50 =56 mg kg −1 ) and gene expression in vivo (ED 50 =67 mg kg −1 ) [9] . We also observed anxiolytic activity of SR9009 in several of these assays ( Fig. 5n-q ). The magnitude of effects we observed with SR9011 and SR9009 was similar to those observed when mice were treated with a benzodiazepine (chlordiazepoxide) ( Supplementary Fig. 5 ). These data, taken together, suggest that pharmacological activation of REV-ERB reduces anxiety-like behaviour while increasing wakefulness rather than decreasing wakefulness, as do most anxiolytic agents. Based on our initial observations of potential anxiolytic activity of SR9011 in chronically dosed mice in metabolic studies, we performed the range of experiments described above using chronically dosed mice. However, we also examined the potential acute anxiolytic effect of SR9011 in the marble-burying assay by administration of 100 mg kg −1 SR9011 followed by initiation of the 30-min assay 30 min after administration. We observed no alteration in marble-burying activity (data not shown), suggesting that chronic administration is required for the anxiolytic activity. 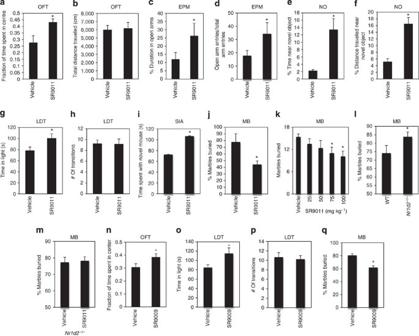Figure 5: REV-ERB regulates anxiety-like behaviour. SR9011 displays anxiolytic activity in a range of behavioural assays. (a) Results from the open-field assay demonstrating that mice administered SR9011 spend a significantly greater amount of time in the centre field during the first 5 min after placing the animals in the apparatus than mice treated with vehicle. (b) SR9011-treated mice display equivalent locomotor activity as vehicle-treated mice in the open-field assay. Results from EPM demonstrates that SR9011-treated mice spend a greater percentage of time exploring the open quadrants (c) and exhibit a greater frequency of open-arm entries (d) than vehicle-treated mice. Results from the novel object (neophobia) assay demonstrating that SR9011-treated mice spend more time near the novel object (e) and travel more distance near the novel object (f) than vehicle-treated mice. Results from the light–dark box assay demonstrating that mice treated with SR9011 spend considerably more time in the light box than vehicle-treated mice (g), while displaying no difference in the total number of transitions between the boxes (h). Results for the SIA assay indicating that mice treated with SR9011 display greater social interaction with a novel mouse than mice treated with vehicle (i). Results from the marble-burying assay demonstrate that SR9011-treated mice bury fewer marbles than vehicle-treated mice (j) and this effect is dose responsive (l). (l)Rev-erbβ−/−mice display more anxiety in the marble-burying assay consistent with data indicating that activation of REV-ERB leads to anxiolytic activity. (m) The REV-ERB agonist, SR9011, does not display anxiolytic activity inRev-erbβ-null mice.Rev-erbβ-null mice were treated with SR9011 in an identical manner as described inland subjected to the marble-burying assay, to examine the potential anxiolytic activity of SR9011. Consistent with the actions of SR9011, a distinct REV-ERB agonist, SR9009, also reduces anxiety-like behaviour in the open-field assay (n), the light–dark transition assay (oandp) and the marble-burying assay (q). Values are mean±s.e.m.,n=12 mice per group for all experiments, except the marble-burying test wheren=8. With the exception ofk, differences between treatment groups (vehicle versus SR) were assessed by a two-tailed Student’st-test with significance *P<0.05. Ink, differences between groups were assessed using one-way ANOVA followed by Tukey’spost hoctest with significance *P<0.05. Figure 5: REV-ERB regulates anxiety-like behaviour. SR9011 displays anxiolytic activity in a range of behavioural assays. ( a ) Results from the open-field assay demonstrating that mice administered SR9011 spend a significantly greater amount of time in the centre field during the first 5 min after placing the animals in the apparatus than mice treated with vehicle. ( b ) SR9011-treated mice display equivalent locomotor activity as vehicle-treated mice in the open-field assay. Results from EPM demonstrates that SR9011-treated mice spend a greater percentage of time exploring the open quadrants ( c ) and exhibit a greater frequency of open-arm entries ( d ) than vehicle-treated mice. Results from the novel object (neophobia) assay demonstrating that SR9011-treated mice spend more time near the novel object ( e ) and travel more distance near the novel object ( f ) than vehicle-treated mice. Results from the light–dark box assay demonstrating that mice treated with SR9011 spend considerably more time in the light box than vehicle-treated mice ( g ), while displaying no difference in the total number of transitions between the boxes ( h ). Results for the SIA assay indicating that mice treated with SR9011 display greater social interaction with a novel mouse than mice treated with vehicle ( i ). Results from the marble-burying assay demonstrate that SR9011-treated mice bury fewer marbles than vehicle-treated mice ( j ) and this effect is dose responsive ( l ). ( l ) Rev-erbβ −/− mice display more anxiety in the marble-burying assay consistent with data indicating that activation of REV-ERB leads to anxiolytic activity. ( m ) The REV-ERB agonist, SR9011, does not display anxiolytic activity in Rev-erbβ -null mice. Rev-erbβ -null mice were treated with SR9011 in an identical manner as described in l and subjected to the marble-burying assay, to examine the potential anxiolytic activity of SR9011. Consistent with the actions of SR9011, a distinct REV-ERB agonist, SR9009, also reduces anxiety-like behaviour in the open-field assay ( n ), the light–dark transition assay ( o and p ) and the marble-burying assay ( q ). Values are mean±s.e.m., n =12 mice per group for all experiments, except the marble-burying test where n =8. With the exception of k , differences between treatment groups (vehicle versus SR) were assessed by a two-tailed Student’s t -test with significance * P <0.05. In k , differences between groups were assessed using one-way ANOVA followed by Tukey’s post hoc test with significance * P <0.05. Full size image We hypothesized that if the effects of SR9011 and SR9009 on reducing anxiety-like behaviour were indeed mediated by REV-ERB, mice lacking the receptor may be more anxious, and that the compound would lack activity in the null mouse. To investigate this, we generated an nr1d2 -null mouse ( Supplementary Fig. 6 ) and examined its activity in the marble-burying assay. As shown in Fig. 5l , these mice displayed greater marble-burying activity consistent with increased anxiety-like behaviour. Furthermore, treatment of the null mice with SR9011 did not alter their behaviour ( Fig. 5m ), indicating that the actions of the compound were at least partially mediated by REV-ERBβ. REV-ERB agonists alter reward-seeking behaviour Many anxiolytics, such as benzodiazepines, are associated with abuse liability related to their positive reinforcing ability. This can be detected in rodents using a conditioned place preference (CPP) assay [29] , [30] , [31] , [32] . We assessed the activity of SR9011 in the CPP assay using an identical dose that displayed anxiolytic activity and found no CPP or aversion ( Fig. 6a ), suggesting that anxiolytics that target REV-ERB may display lower abuse potential than benzodiazapenes. Interestingly, we previously noted that administration of REV-ERB agonists results in loss of wheel-running activity even though locomotor behaviour was not affected [9] . The EEG data described above confirm this observation, demonstrating that the mice are wakeful and exhibit locomotor activity during periods where we have observed loss of wheel-running activity. This suggested that the REV-ERB agonists might be altering motivation to run on the wheel. Wheel running in rodents is a well-defined rewarding behaviour [33] , [34] , [35] and thus we hypothesized that REV-ERB agonists may be interfering with the central reward pathway. To investigate this, we performed an additional CPP assay where we compared the effect of administration of cocaine alone with coadministration of SR9011 with cocaine. As illustrated in Fig. 6b , a clear condition place preference was observed with cocaine that was inhibited by coadministration of SR9011. These data suggest that REV-ERB agonists suppress the rewarding behaviour associated with wheel running and cocaine, yet the agonist by itself does not induce aversive behaviour. 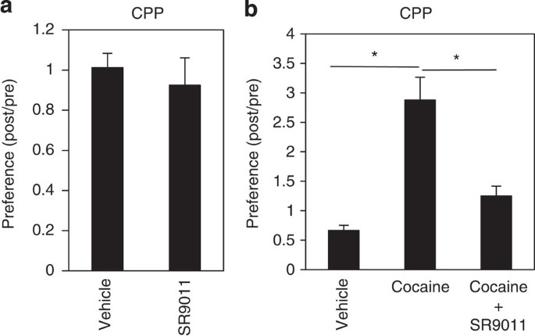Figure 6: REV-ERB activation alters reward-seeking behaviour. (a) Results from a CPP assay indicating lack of CPP or aversion activity of SR9011. Differences between treatment groups (vehicle versus SR) were assessed by a two-tailed Student’st-test with significance *P<0.05. (b) Results of a CPP assay indicating that SR9011 coadministration inhibits the CPP displayed by cocaine. Differences between groups were assessed using one-way ANOVA followed by Tukey’spost hoctest with significance *P<0.05. Values are mean±s.e.m.,n=12 mice per group for all experiments. Figure 6: REV-ERB activation alters reward-seeking behaviour. ( a ) Results from a CPP assay indicating lack of CPP or aversion activity of SR9011. Differences between treatment groups (vehicle versus SR) were assessed by a two-tailed Student’s t -test with significance * P <0.05. ( b ) Results of a CPP assay indicating that SR9011 coadministration inhibits the CPP displayed by cocaine. Differences between groups were assessed using one-way ANOVA followed by Tukey’s post hoc test with significance * P <0.05. Values are mean±s.e.m., n =12 mice per group for all experiments. Full size image Mice harbouring a mutation in the clock gene have been shown to display a behavioural profile similar to human mania [25] . Furthermore, polymorphisms in the human gene encoding REV-ERBα ( NR1D1 ) are associated with bipolar disorder [21] . As previously discussed, REV-ERB agonists would be expected to reduce clock expression levels and may mimic the effect observed in these mice. According to the Diagnostic and Statistical Manual of Mental Disorders, Fifth Edition, a manic episode in humans is characterized by the presence of at least three symptoms of seven, which include reduced anxiety (elated mood) and increased wakefulness, leading us to consider whether the REV-ERB agonists may be inducing a behavioural profile similar to mania. Clearly, we observe reduced anxiety ( Fig. 5 ) and increased wakefulness ( Figs 1 and 3 ). However, we do not observe an effect on depression-like behaviour in a tail-suspension assay ( Supplementary Fig. 7 ) and we also observe a distinctly opposite effect on the reward value of cocaine ( Fig. 6b ). SR10067 is a novel REV-ERB agonist with high affinity SR9011 and SR9009 were the first synthetic REV-ERB agonists developed with sufficient pharmacokinetic properties, to be used as in vivo chemical tools [9] . However, they exhibit relatively low potency for the receptor with IC 50 ’s of ~700 nM [9] . We hypothesized that if activation of REV-ERB with synthetic agonists did indeed lead to the wakefulness and anxiolytic effects, development of higher-affinity REV-ERB agonists with either equivalent or improved pharmacokinetic properties should yield improvements in the in vivo potency. To test this hypothesis, we evaluated a synthetic REV-ERB agonist (SR10067) derived from extensive modification of the SR9009/SR9011 scaffold [36] , [37] ( Fig. 7a and Supplementary Figs 8 and 9 ) that displays substantially greater potency than SR9011 and SR9009 in vitro . The potency of SR10067 is considerably better than SR9011 and SR9009 in the Gal4DBD-REV-ERB ligand-binding domain cotransfection assay (SR10067: REV-ERBα IC 50 =170 nM, REV-ERBβ IC 50 =160 nM ( Fig. 7b ) versus SR9011: REV-ERBα IC 50 =670 nM, REV-ERBβ IC 50 =800 nM [9] ). Potency of SR10067 was also considerably better in a cotransfection assay using full-length REV-ERBα along with the BMAL1 promoter luciferase reporter (SR10067 IC 50 =140 nM ( Fig. 8c ) versus SR9011 IC 50 =620 nM [9] ). SR10067 displayed no significant activity at any other nuclear receptor ( Fig. 7e ) or a range of other receptors, ion channels and transporters assessed in the NIMH Psychoactive Drug Screening Program ( Supplementary Table 1 . Assessment of plasma and brain concentrations of SR10067 1 and 6 h after i.p. injection (30 mg kg −1 ) revealed that levels of the compound remain above the IC 50 for the receptor 6 h after administration ( Fig. 7d ). As a marker of in vivo efficacy of REV-ERB agonists, we previously demonstrated that a single injection of SR9011 or SR9009 suppressed the circadian rhythm of Npas2 gene expression in the mouse hypothalamus [9] , and when we performed this experiment with SR10067 we observed similar results ( Fig. 7f ). Synthetic REV-ERB agonists also suppress circadian wheel-running activity after a single injection [9] and this was observed with SR10067. As illustrated in Fig. 8a,b , administration of SR10067 at various concentrations yielded a dose-dependent effect on reduction in nocturnal wheel-running activity as indicated in the actograms. The ED 50 for suppression of wheel-running activity was 20 mg kg −1 ( Fig. 8b ), which is more potent than that described for SR9011 (56 mg kg −1 ) [9] and is consistent with the improved potency of SR10067 in the REV-ERB transcriptional assays. SR10067 induced wakefulness and reduced SWS and REM sleep when injected at ZT6, similar to what was observed with SR9011 and SR9009 ( Fig. 8c ). The effect of SR10067 on sleep architecture was also similar to what was observed with SR9011 and SR9009, with increased number of episodes of SWS with decreased duration and decreased number of episodes and duration of REM sleep ( Fig. 9 ). No effect on EEG power was observed ( Supplementary Fig. 1C ). SR10067 also induced locomotion when administered into mice at ZT6 in a manner similar to SR9009 and SR9011, consistent with an increase in wakefulness ( Fig. 8d ). The anxiolytic activity of SR10067 was assessed in the marble burying anxiety assay and SR10067 displayed superior potency than SR9011 (ED 50 of 12versus 61 mg kg −1 ) ( Fig. 8e ). This fivefold improvement in in vivo anxiolytic potency compares favourably with the in vitro improvement in potency (four- to fivefold) when comparing SR10067 with SR9011. These data clearly suggest that the anxiolytic activity is mediated by activation of REV-ERB given that two synthetic REV-ERB selective agonists, with distinct chemical structures, display anxiolytic activity that correlates to their relative activity at REV-ERB. 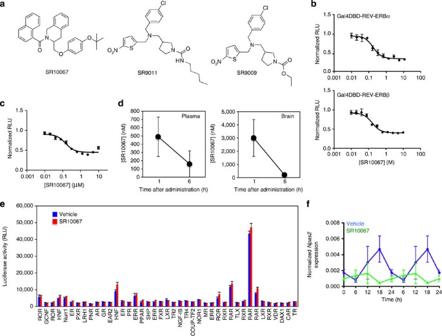Figure 7: Identification of SR10067 as a highly potent synthetic REV-ERB agonist. (a) Chemical structure of the synthetic REV-ERB agonist SR10067 compared with SR9011 and SR9009. (b) Results from a Gal4-REV-ERB/Gal4 UASX5 luciferase reporter co-transfection assay in HEK293 cells displaying the potent REV-ERB agonist activity of SR10067. (c) Results from a co-transfection assay in HEK 293 cells with full-length REV-ERBα and aBMAL1promoter-driven luciferase reporter displaying the potent agonist activity of SR10067. (d) Plasma and brain concentrations of SR10067 2 h following i.p. injection of 30 mg kg−1of the compound. The 6-h value for SR10067 in the brain is 150±20 nM. (e) Nuclear receptor specificity assay illustrating lack of activity of SR10067 on a wide range of nuclear receptors. The format of the assay was a co-transfection assay with Gal4 DNA-binding domain–nuclear receptor fusions in HEK293 cells as previously described (see Methods). SR10067 was tested at 20 μM. Error bars indicate mean±s.e.m. andn=3. There were no statistical differences between vehicle and drug treatment in any of the assays shown as assessed by a Student’st-test (unpaired two-tailed). (f) Normalized (toGapdh) expression ofNpas2mRNA isolated from the hypothalamic of mice injected with 30 mg kg−1of SR10067 (i.p. at ZT0) demonstrating a SR10067-dependent alteration in the circadian rhythm of expression. Expression was monitored over 24 h and the results are double plotted.n=5. *P<0.05. Mean±s.e.m. Figure 7: Identification of SR10067 as a highly potent synthetic REV-ERB agonist. ( a ) Chemical structure of the synthetic REV-ERB agonist SR10067 compared with SR9011 and SR9009. ( b ) Results from a Gal4-REV-ERB/Gal4 UASX5 luciferase reporter co-transfection assay in HEK293 cells displaying the potent REV-ERB agonist activity of SR10067. ( c ) Results from a co-transfection assay in HEK 293 cells with full-length REV-ERBα and a BMAL1 promoter-driven luciferase reporter displaying the potent agonist activity of SR10067. ( d ) Plasma and brain concentrations of SR10067 2 h following i.p. injection of 30 mg kg −1 of the compound. The 6-h value for SR10067 in the brain is 150±20 nM. ( e ) Nuclear receptor specificity assay illustrating lack of activity of SR10067 on a wide range of nuclear receptors. The format of the assay was a co-transfection assay with Gal4 DNA-binding domain–nuclear receptor fusions in HEK293 cells as previously described (see Methods). SR10067 was tested at 20 μM. Error bars indicate mean±s.e.m. and n =3. There were no statistical differences between vehicle and drug treatment in any of the assays shown as assessed by a Student’s t -test (unpaired two-tailed). ( f ) Normalized (to Gapdh ) expression of Npas2 mRNA isolated from the hypothalamic of mice injected with 30 mg kg −1 of SR10067 (i.p. at ZT0) demonstrating a SR10067-dependent alteration in the circadian rhythm of expression. Expression was monitored over 24 h and the results are double plotted. n =5. * P <0.05. Mean±s.e.m. 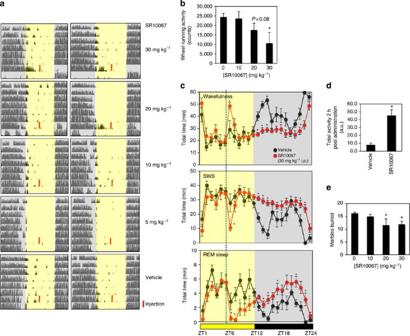Figure 8: SR10067 alters sleep architecture and anxiety-like behaviour. (a) Actograms from wheel-running cages demonstrating the effect of SR10067 injection (red bars, i.p. various concentrations) on wheel-running activity in mice. (b) Assessment of the dose dependence of inhibition of wheel-running activity in mice during the entire dark phase following administration of SR10067.n=6–8 mice per group. (c) Assessment of the effect of SR10067 on wakefulness in mice. Wakefulness, SWS and REM sleep was monitored by EEG as indicated inFigs 1and2. Mice were injected with SR10067 (30 mg kg−1, i.p.) or vehicle at ZT6.n=8 mice. (d) Locomotor telemetry data indicating an increase in movement of mice during the period 2 h after ZT6 injection of SR10067 (30 mg kg−1).n=6 mice. (e) Results from the marble-burying assay demonstrating that SR10067 dose dependently reduces anxiety-like behaviour in the marble-burying assay.n=8 mice. Values are mean±s.e.m. Ind, differences between treatment groups (vehicle versus SR) were assessed by a two tailed Student’st-test () with significance *P<0.05. Inbande, differences between groups were assessed using one-way ANOVA followed by Tukey’spost hoctest with significance *P<0.05. Inc, potential differences between treatments were assessed by repeated-measures two-way ANOVA followed by Bonferronipost hoctest with significance *P<0.05. Full size image Figure 8: SR10067 alters sleep architecture and anxiety-like behaviour. ( a ) Actograms from wheel-running cages demonstrating the effect of SR10067 injection (red bars, i.p. various concentrations) on wheel-running activity in mice. ( b ) Assessment of the dose dependence of inhibition of wheel-running activity in mice during the entire dark phase following administration of SR10067. n =6–8 mice per group. ( c ) Assessment of the effect of SR10067 on wakefulness in mice. Wakefulness, SWS and REM sleep was monitored by EEG as indicated in Figs 1 and 2 . Mice were injected with SR10067 (30 mg kg −1 , i.p.) or vehicle at ZT6. n =8 mice. ( d ) Locomotor telemetry data indicating an increase in movement of mice during the period 2 h after ZT6 injection of SR10067 (30 mg kg −1 ). n =6 mice. ( e ) Results from the marble-burying assay demonstrating that SR10067 dose dependently reduces anxiety-like behaviour in the marble-burying assay. n =8 mice. Values are mean±s.e.m. In d , differences between treatment groups (vehicle versus SR) were assessed by a two tailed Student’s t -test () with significance * P <0.05. In b and e , differences between groups were assessed using one-way ANOVA followed by Tukey’s post hoc test with significance * P <0.05. In c , potential differences between treatments were assessed by repeated-measures two-way ANOVA followed by Bonferroni post hoc test with significance * P <0.05. 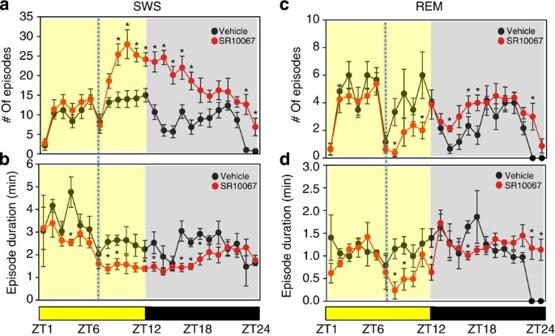Figure 9: Administration of SR10067 alters sleep architecture. Effect of SR10067 administered at ZT6 (analysis of data fromFig. 9c) on SWS (number of episodes (a) and episode duration (b)) and on REM sleep (number of episodes (c) and episode duration (d)). Potential differences between treatments were assessed by repeated-measures two-way ANOVA followed by Bonferronipost hoctest with significance *P<0.05. Full size image Figure 9: Administration of SR10067 alters sleep architecture. Effect of SR10067 administered at ZT6 (analysis of data from Fig. 9c ) on SWS (number of episodes ( a ) and episode duration ( b )) and on REM sleep (number of episodes ( c ) and episode duration ( d )). Potential differences between treatments were assessed by repeated-measures two-way ANOVA followed by Bonferroni post hoc test with significance * P <0.05. Full size image The mammalian clock maintains the circadian rhythm that is essential for normal physiological function. Mutation of components of the clock alters normal physiological processes at multiple levels including sleep, metabolism, behaviour and so on [7] , [38] , [39] . Alteration of the normal circadian rhythm in humans due to shift work or experimental manipulation alters the metabolic and mental health of individuals. In addition, circadian disruption is commonly noted in a range of psychiatric disorders including anxiety, schizophrenia and depression [12] , [13] , [14] , [15] . It has been unclear whether molecular components of the mammalian clock could be targeted for development of therapeutics, and recently small molecule regulators of the core clock have been discovered and developed [10] , [40] . Small molecule inhibitors [41] and activators [42] of CRY have been discovered and they regulate the circadian rhythm in cell lines, but none have progressed to evaluation in animal models to determine their potential utility for treatment of disease. It has been suggested that REV-ERB be considered as a core component of the clock, as mice lacking both REV-ERBα and REV-ERBβ are arrhythmic [4] . Our recent study demonstrated that synthetic REV-ERB agonists alter the circadian rhythm and improve the metabolic profile in mouse models of metabolic disease. Here we show that pharmacological targeting of the core clock has further value, demonstrating the ability of REV-ERB agonists to modulate sleep and emotional behaviour. In mice treated with various REV-ERB agonists, we observed alterations in patterns of sleep–wakefulness, sleep architecture and the level of anxiety. Clock genes have been demonstrated to play an important role in regulation of sleep. Bmal1 -null mice display increased sleep and this sleep displays increased fragmentation [43] . Clock mutant mice display reduced non-REM sleep, while Cry1/Cry2 -null mice display an increase in non-REM sleep [44] , [45] . Npas2 -null mice as well as Per -null mice also display alterations in the patterns of sleep [46] , [47] , [48] . Given the role that REV-ERB plays in regulation of these genes, we believed there would be an effect of pharmacological modulation of REV-ERB activity on sleep. All of the studies examining the effect of clock genes on sleep are genetic loss of function studies and not pharmacological studies; thus, we were not sure what to expect with the first examination of pharmacological targeting of a clock gene on sleep. Administration of REV-ERB agonists stimulates wakefulness and suppresses sleep. This effect is acute, which is consistent with the short half-life of the compounds, and the mice return to a normal sleep pattern within ~12 h. The lack of effect on long-term circadian behaviour is consistent with our previous data indicating that REV-ERB agonists only transiently altered circadian wheel-running behaviour followed to a return to a normal circadian rhythm [9] . Sleep disorders affect ~70 million individuals in the United States and therapeutics such as the REV-ERB agonists that induce wakefulness while also reducing anxiety should be examined for treatment of shift work–sleep disorder and sleep apnoea. Previously, we demonstrated that REV-ERB agonists increase the metabolic rate and are quite effective in increasing oxidative metabolism in skeletal muscle [9] , [11] . This would probably be associated with an increase in core body temperature; however, a recent study also demonstrated that Ucp1 is a direct REV-ERB target gene, and that in brown adipose tissue loss of REV-ERBα leads to a decrease in thermogenic brown adipose tissue activity [49] . Thus, it was unclear what the summation of effect of pharmacological activation of REV-ERB on core body temperature would be. We observed that pharmacological activation of REV-ERB led to a transient increase in core body temperature when administered at ZT6, but the elevation of temperature was not equivalent to that observed during normal wakefulness in the dark period. Interestingly, in the transition to darkness when mice administered REV-ERB agonists displayed sleep recovery, they also displayed an increase in body core temperature that was indistinguishable from mice administered vehicle that displayed normal wakefulness. Alterations in sleep and wakefulness have been associated with changes in cellular energetics [50] , and although modulation of REV-ERB activity may indeed alter patterns of sleep and wakefulness by altering cellular energetics, we observed that these can be uncoupled, at least in terms of gross measurements of body core temperature. Even more intriguing is our observation that REV-ERB agonists reduced anxiety-like behaviour in mice in an array of behavioural assays that are models of generalized anxiety disorder and social anxiety disorder [51] . Although there is data to suggest that the mammalian clock is involved in anxiety, there have been no chemical tools available until recently, to effectively address the potential to alter the central anxiety pathways by altering the clock. Anxiety disorders are among the most common mental disorders and nearly 30% of individuals will be directly affected by an anxiety disorder at some point in their lifetime; thus, these disorders significantly burden our society [52] , [53] , [54] . Given the predominance of anxiety disorders in our society, there continues to be a focus on development of novel anxiolytic agents with improved efficacy and/or side-effect profiles. Clearly, the pharmacological profile of these compounds is paradoxical, given their ability to combine anxiolytic activity with increased wakefulness, which could offer a clear clinical advantage under many circumstances. Drugs that typically increase arousal also increase anxiety (forexample, cocaine and amphetamines), while drugs that decrease anxiety decrease arousal (for example, benzodiazepines and ethanol) [55] . Exceptions to this profile include nicotine [56] and Neuropeptide S [57] , but the pharmacological profile of REV-ERB agonists and their ability to target the clock appear to be distinct from these pathways. It is also important to note that SR9011 inhibited the condition place preference associated with cocaine-induced reward without itself inducing aversion. Our data indicating that mice treated with various REV-ERB agonists failed to wheel run during periods when they were awake led us to hypothesize that there may be suppression of reward-seeking behaviour. Drug addiction clearly has a circadian component [58] and mice with mutations in clock genes such as Per1 , Per2 , Clock and Npas2 have altered responsiveness to the reward associated with cocaine, morphine and/or alcohol [25] , [59] , [60] , [61] . Thus, it is quite reasonable to expect that a small molecule regulator of the clock would modulate reward-seeking behaviour. These data suggest that modulation of the clock by small molecule drugs, such as REV-ERB agonists, may have utility in treatment of addiction. Using a variety of approaches including mouse genetic models, epidemiology, clinical research, circadian rhythms and the underlying molecular clock mechanism have been associated with a variety of disorders. With recent chemical biology approaches, it has become possible to target certain components of the clock and begin to investigate whether pharmacological modulation of clock function and the circadian rhythm may offer an approach to treat human disease. In summary, our data indicate that pharmacological targeting of the clock holds promise for treatment of disorders associated with anxiety and sleep disorders, as well as addiction. Synthesis and preparation of SR9011 and SR9009 SR9011 and SR9009 were prepared as previously described [9] . Synthesis and preparation of SR10067 DL-(1,2,3,4-tetrahydroisoquinolin-3-yl)methanol . DL-1,2,3,4-tetrahydroisoquinoline-3-carboxylic acid (3.54 g, 20 mmol) was added portion wise to a suspension of LiAlH 4 (3.04 g, 80 mmol) in tetrahydrofuran (150 ml) at 0 °C under argon. The reaction mixture was heated under reflux for 16 h. It was then cooled to 0 °C, and water (3 ml), 15% aqueous NaOH (3 ml) and water (9 ml) were added under stirring. The precipitate was then filtered and washed with diethyl ether (3 × 100 ml). The solvent was removed under vacuum and the product obtained as brown microcrystals (76%) was used in the next step without further purification. 1H NMR (400 MHz, CDCl 3 ): δ (p.p.m.) 7.18–7.05 ( m , 3H), 7.06–7.00 ( m , 1H), 4.05 ( s , 2H), 3.76 (dt, J =10.9, 3.1 Hz, 1H), 3.51 (dd, J =10.8, 7.9 Hz, 1H), 3.05 (ddq, J =11.3, 7.4, 3.7 Hz, 1H), 2.69 (dt, J =16.3, 3.4 Hz, 1H), 2.57 (dd, J =16.4, 10.8 Hz, 1H); 13C NMR (100 MHz, CDCl3): δ (p.p.m.) 135.6, 134.1, 129.4, 126.4, 126.2, 126.0, 65.7, 55.2, 48.0, 31.1; high-resolution mass spectroscopy (HRMS) calculated for C 10 H 13 NO (M+H)+: 164.1069, found: 164.1051. (3-(Hydroxymethyl)-3,4-dihydroisoquinolin-2(1H)-yl)(naphthalen-1-yl)methanone . To a solution of DL-(1,2,3,4-Tetrahydroisoquinolin-3-yl)methanol (0.816 g, 55 mmol) in dicholoromethane was added 1-naphthoyl chloride (0.908 ml, 6 mmol), and triethylamine (1.36 ml, 10 mmol) and the mixture was stirred for 12 h. The reaction mixture was washed with HCl (2 N), saturated sodium bicarbonate solution and brine. The organic phase was separated, dried over anhydrous MgSO 4 and the solvent was removed under reduced pressure. The residue was then purified by flash chromatography on silica gel (ethyl acetate/hexanes) to give the title compound as light-brown microcrystals (78.8%). 1H NMR (400 MHz, Chloroform-d) δ (p.p.m.) 1 H NMR (400 MHz, CDCl 3 ): (mixture of rotamers) δ (p.p.m.) 8.05 ( t , J =9.5 Hz, 0.6H), 7.98–7.76 ( m , 2.4H), 7.64–7.44 ( m , 3.4H), 7.37 (dd, J =20.3, 7.5 Hz, 1H), 7.25–7.17 ( m , 2H), 7.16–7.01 ( m , 1H), 6.75–6.62 ( m , 0.5H), 5.69–5.58 ( m , 0.5H), 5.33–5.20 ( m , 0.5H), 4.59–4.00 ( m , 2H), 3.96–3.72 ( m , 1H), 3.64–3.48 ( m , 0.5H), 3.30–3.10 ( m , 1H), 3.04–2.79 ( m , 1H), 2.68–2.51 ( m , 0.5H); 13 C NMR (100 MHz, CDCl 3 ): (mixture of rotamers) δ (p.p.m.) 172.12, 171.33, 134.57, 134.50, 133.60, 133.35, 132.75, 131.51, 129.58, 129.53, 129.45, 129.32, 129.09, 128.92, 128.62, 128.55, 128.49, 128.33, 127.57, 127.49, 127.13, 127.08, 126.89, 126.74, 126.71, 126.65, 126.58, 126.49, 126.45, 125.70, 125.54, 125.37, 125.33, 125.16, 124.76, 124.48, 123.77, 63.81, 63.63, 61.66, 61.22, 54.39, 51.36, 51.32, 46.36, 42.05, 41.31, 41.22, 30.23, 30.07, 29.86, 29.82; HRMS calculated for C 21 H 19 NO 2 (M+H)+: 318.1489, found: 318.1491. (3-((4-(Tert-butoxy)phenoxy)methyl)-3,4-dihydroisoquinolin-2(1H)-yl)(naphthalen-1-yl)methanone . To a solution of (3-(hydroxymethyl)-3,4-dihydroisoquinolin-2(1H)-yl)(naphthalen-1-yl)methanone (0.317 g, 1 mmol), triphenylphosphine (0.288 g, 1.1 mmol) and 4-(tert-butoxy)phenol (0.166 g, 1 mmol) in dry toluene (2 ml) at 0 °C was added diisopropyl azodicarboxylate (0.216 ml, 1.1 mmol) dropwise. The mixture was stirred at ambient temperature overnight. The solvent was evaporated and the residue was then purified by flash chromatography on silica gel (ethyl acetate/hexanes) to give the title compound as a white microcrystals (50%). 1 H NMR (400 MHz, CDCl 3 ): (mixture of rotamers) δ 8.23–8.12 ( m , 0.5H), 7.98–7.82 ( m , 2H), 7.76–7.41 ( m , 4H), 7.34–7.06 ( m , 4H), 7.02–6.83 ( m , 2H), 6.79–6.63 ( m , 2H), 6.50–6.42 ( m , 0.5H), 5.82–5.52 ( m , 1H), 4.60–4.36 ( m , 1H), 4.35–4.10 ( m , 2H), 3.92 (dt, J =12.6, 9.5 Hz, 0.5H), 3.70 (ddd, J =31.9, 9.8, 6.1 Hz, 0.5H), 3.35 (dd, J =16.3, 6.3 Hz, 0.5H), 3.31–3.05 ( m , 1H), 2.84–2.61 ( m , 0.5H), 1.36–1.25 ( m , 9H); 1 H NMR (400 MHz, d 6 -DMSO, 110 °C): δ 8.0 ( d , 2H), 7.8 (br s, 1H), 7.62–7.58 ( m , 4H), 7.2 (br s, 3H), 7.0–6.5 (br m , 4H), 5.5 (br s, 1H), 4.5–3.7 ( m , 4H), 3.3–2.8 ( m , 2H), 1.3 ( s , 9H); 13 C NMR (100 MHz, CDCl 3 ): (mixture of rotamers) δ (p.p.m.) 171.11, 171.07, 170.58, 154.88, 154.50, 154.30, 149.13, 149.10, 148.93, 134.38, 132.83, 129.41, 127.02, 126.91, 126.87, 125.56, 125.53, 125.47, 125.27, 114.86, 114.72, 114.51, 114.37, 78.31, 78.29, 78.21, 67.16, 66.79, 52.57, 52.03, 47.81, 41.28, 41.20, 34.79, 30.73, 28.85, 28.79, 28.77, 22.78, 22.08, 14.26; 13 C NMR (100 MHz, d 6 -DMSO, 110 °C): 169.8, 154.5, 149.5, 135.1, 133.6, 129.2, 128.7, 127.2, 126.7, 126.6, 125.6, 124.8, 124.2, 115.4, 77.8, 67.8, 52.3, 30.1, 29.0; HRMS calculated for C 31 H 31 NO 3 (M+H)+: 466.2376, found: 466.2373. Pharmacokinetic studies Pharmacokinetic studies were performed as previously described [1] . Co-transfection assays Co-transfection assays were performed as previously described in HEK293 cells (Gal4cotransfection assay) or in HepG2 cells (full-length nuclear receptors) [1] . Cells were recently obtained from the ATCC (within four passages) and monitored for mycoplasma contamination. Mice C57BL6 and Balb/c male mice were obtained from the Jackson Laboratories (Bar Harbor, ME). All the procedures were conducted in the Scripps or SLU vivarium, which are fully accredited by the Association for Assessment and Accreditation of Laboratory Animal Care, and were approved by the Scripps Institutional Animal Care and Use Committee and the SLU Institutional Animal Care and Use Commitee. All experiments were conducted at 22–23 °C. Compound administration For all experiments, 8-week-old C57BL6/J or Balb/c male mice were administered doses of SR9011 or SR9009 100 mg kg −1 (i.p., b.i.d.) for 3–10 days for behavioural assays. See Supplementary Fig. 5 for a schematic of the dosing and testing regimen. For twice per day dosing, dosing was performed at ZT0 and ZT12. For the first testing regimen open-field assay, light–dark transfer assay, marble-burying assay and tail-suspension assays were performed after 3, 5, 8 and 10 days of dosing, respectively. These assays were typically performed 1–2 h after the ZT12 injection under red light. However, the open-field and marble-burying assays were also performed at ZT6–8 and under normal light conditions with no distinction in efficacy of SR9011, indicating that the anxiolytic action was not time of day dependent. For the second regimen, the novel object and EPM assays were performed after 3 and 5 days of twice per day dosing, respectively, at ZT 6–8 under normal light conditions. Initially, multiple assays were performed in this manner so as to allow the same cohort of animals to be examined in multiple assays. However, if single assays were run, the identical dosing regimen was employed for consistency. The CPP and SIA assay were performed after 5 days of dosing. SR10067 was administered at various doses as indicated in the figure legends. The specifics of administration of compounds for sleep studies is indicated in the figures/figure legends. Formulation of the REV-ERB agonists was performed as previously described [9] . For studies where LiCl was used, mice were provided LiCl in drinking water (600 mg l −1 ), while control mice received normal water for 10 days before initiation of the study. The LiCl drinking water was maintained during the study. For studies using cocaine, Cocaine hydrochloride (National Institute on Drug Abuse) was dissolved in sterile 0.9% saline solution. Mice were administered 10 mg kg −1 cocaine in the CPP studies and doses as indicated in the figure in the EEG studies. Gene targeting Standard gene targeting procedures [62] were used to generate mice with floxed alleles at the Rev-erbβ locus on a C57BL6/6J background. The floxed Rev-erbβ mice were generated at the transgenic core at the Pennington Biomedical Research Center in Baton Rouge, LA. The strategy for generation of the mice is shown in Supplementary Fig. 7A . For generation of the germ line-deleted strain, the floxed Rev-erbβ mice were mated with Ella-Cre mice. Open-field and neophobia assays Mice were handled 2 min daily for 3 days before testing their spontaneous locomotor activity and reactivity to novelty in an activity chamber. The chamber where the mice were assessed is a rectangle (37 cm × 57 cm) that is divideded into nine virtual zones of identical size (~12 cm × 19 cm zones). The open-field assay was initiated by placing the mice in the centre of the chamber. The locomotor activity was monitored by a video camera mounted on the ceiling and a computerized tracking system (Ethovision 1.90, Noldus IT, Wageningen, The Netherlands) recorded the total distance moved, speed and percentage of time spent in each zone. Time occupied in the centre zone (~12 cm × 19 cm) and latency to enter the centre zone was assessed for the open-field assay as well as total distance travelled. For the neophobia assay, mice that had already been assessed in the open-field assay and thus familiar with the chamber were placed into the centre of the chamber to which a novel object had been fixed. The novel object was a 7 black rubber stopper placed at the top centre of the chamber (zone 2 if one considers the activity box consisting of three rows of three zones) and the reactivity of the animal towards the object was measured. Zone 2 was considered near the novel object and time spent in this zone was scored. The floor of the arena and the object were washed after each test, with 70% ethanol solution to remove odours left by previous subjects. Elevated plus maze Anxiety-like behaviour of mice were evaluated using the EPM test. The EPM consisted of two opposing open arms (45 cm × 10 cm) and two closed arms (45 cm × 10 cm × 50 cm) that extended from a central platform (10 cm × 10 cm) elevated 65 cm above the floor. Mice were placed individually on the central platform facing a closed arm and were allowed to freely explore the maze for 5 min. The behaviour of each mouse was monitored using a video camera and the movement of the mice automatically registered and analysed with a computerized tracking system (Ethovision 1.90, Noldus IT). Entry into an arm was defined as entry of all four paws into the arm. Total distance moved, speed, time spent in the open and closed arms, number of times the animal entered each type of arm and latency before entering an open arm were measured. Animal’s grooming, stretching and rearing behaviours, as well as the exploration outside the maze (head dipping), were measured. The floor of the EPM was washed after each testing with 70% ethanol solution to remove odours left by previous subjects. Marble-burying assay The marble-burying test is used to assess anxiety-like behaviour in a less vision-dependent manner than other available tests such as the EPM and light/dark transfer tests. Mice were placed individually in a standard mouse cage containing bedding that is 5 cm in depth, with 20 small marbles arranged in 4 evenly spaced rows of 5 on top of the bedding material as previously described [57] . After 30 min, mice were removed and the number of marbles buried (at least two of three covered by bedding) is determined. Increased marble burying is associated with increased anxiety-like behaviour in tests of anxiety medications. Light–dark box assay The light–dark transfer procedure has been used to assess anxiety-like behaviour in mice by capitalizing on the conflict between exploration of a novel environment and the avoidance of a brightly lit open field [57] . The apparatus is a rectangular box made of Plexiglas divided by a partition into two environments. One compartment (14.5 × 27 × 26.5 cm) is dark (8–16 lux) and the other compartment (28.5 × 27 × 26.5 cm) is highly illuminated (600–800 lux) by a 60-W light source located above it. The compartments are connected by an opening (7.5 × 7.5 cm) located at floor level in the centre of the partition. The time spent in the light compartment was used as a predictor of anxiety-like behaviour, that is, a greater amount of time in the light compartment was indicative of decreased anxiety-like behaviour. Mice were placed in the dark compartment to start the 5-min test. Conditioned place preference assay Studies were conducted using a three-compartment apparatus with two equal-sized chambers (17 × 12.7 × 12.3 cm) separated by a neutral gray chamber (8.5 × 12.7 × 12.3 cm) (ENV-3013; Med Associates, St Albans, VT). The large compartments differed in the wall colour (black or white) and flooring (wire bars or wire mesh), and were separated from the centre gray compartment by sliding doors. Mice were first assessed for baseline preference across two 30-min sessions. Each animal was placed in the centre gray chamber and permitted to freely move through the chambers. Time spent in each chamber was recorded using Med PC software. Based on the time spent in either the white or black chamber during the baseline sessions the non-preferred chamber was assigned as the drug-paired chamber, while the preferred chamber was paired with saline. Mice were subsequently trained across 6 consecutive days. For each session, animals were injected with either the drug or vehicle 15 min before being confined to the assigned white or black chamber for 30 min. Injection and chamber pairings were counterbalanced across training sessions. On the final test day, mice were placed in the centre gray compartment and permitted to freely move throughout the apparatus for 30 min. The time spent in each chamber was recorded as above and the data from the test day were compared with the baseline level to obtain a preference score (post training/pre training). Electroencephalogram EEG analysis was performed as previously described [63] , [64] , [65] , [66] . EEG data are recorded from stainless steel screw electrodes implanted on the frontal and parietal bone over the hippocampus (coordinates: 2.0 mm posterior and 2.0 mm lateral to the bregma according to The Mouse Brain in Stereotaxic Coordinates from Franklin and Paxinos, 1977), and under general anaesthesia (1–1.5% isoflurane). A fourth EEG electrode is implanted over the cerebellum, which is used to ground the animal to reduce signal artefacts. Insulated leads from the EEG electrodes are crimped to male pins (220-P02) and then cemented to the skull with dental acrylic. Following surgical implantation, mice are allowed 1–2 weeks to recover before the study. To record EEG, mice are connected to commutators (PlasticOne) with flexible recording cables allowing them unrestricted movements within the cage and habituated to the recording cages for 48 h. Compounds were administered and recording was continued for another 48 h. The EEG and electromyography signals were amplified in a Grass Model 7D polygraph in a frequency range of 0.3 to 10 KHz. The EEG and EMG are displayed on a computer monitor and stored with a resolution of 128 Hz in the hard drive of a computer for the offline analysis of the vigilance states and spectral analysis using software supplied by Kissei Comptec. The polygraphic results are analysed semi-automatically by 15-s epochs and classified as W, SWS and REM sleep. The total time of these vigilance states is calculated in periods of 1 h. The number and duration of the individual W, SWS and REM sleep episodes are evaluated. In addition to standard sleep analysis, EEG spectral analysis in the different states of vigilance is performed by Fourier fast transformer analysis using 4-s epochs instead of the 15-s epochs. Tail suspension test The tail suspension test was carried out essentially as previously described by Steru et al. [67] Mice were allowed to acclimatize to the holding room for 30 min before the behavioural procedure. One hour after the final administration of vehicle or SR9011, mice were individually suspended by the tail from each of the hooks of the tail suspension test apparatus using adhesive tape placed about one-third away from the tip of the tail. Immobility duration was recorded for 6 min after 1 min of acclimatization. Mice were considered immobile only when they hung passively and completely motionless. The duration of immobility during the 6-min test period was automatically recorded by a camera and stored on a computer equipped with EthoVision XT software. Telemetric assessment of locomotor activity and core body temperature The Physiotel TA-F10 transmitters (Data Sciences International, USA) were surgically implanted to the peritoneal cavity of mice under constant general isofluorane anaesthesia (1–1.5%). The implanted mice were allowed to recover for 7 days before the telemetric recordings started. Post-surgical care included antibiotic treatment (enrofloxacin 2.5–5 mg kg −1 , subcutaneously) for 5 days and management of pain with Rimadyl tablets (2 mg). The locomotor and temperature signals were wirelessly collected by a radio receiver (PhysioTel RPC-1, Data Sciences International) placed on the bottom of each mouse cage. The signals were transferred to data matrixes (PhysioTel Multiplus Analog Adaptor Model DL-10, Data Sciences International) that amplified and converted the analogical signals to digital data that was acquired continuously in real time at 250 Hz, using the computer-based Dataquest ART acquisition software (Data Sciences International). The acquired data were analysed using Neuroscore (Data Sciences International) and the sum of arbitrary counts of locomotor activity obtained for the 2 h following vehicle or compound administration was presented. Core body temperature was monitored over 24 h. Social interaction assay C57BL/6J mice were used in this experiment. They were administered 100 mg kg −1 SR9011 or vehicle i.p. b.i.d. for 5 days and were tested in the social interaction test 1 h following the final injection. This test was originally developed to model in mice aspects of autism spectrum disorders in humans [68] , [69] and has been used widely by behavioural neuroscientists [70] . In addition, the SIA assay has been used as a model for social anxiety disorder [51] . The social interaction apparatus is a rectangular, three-chambered Plexiglas box, with each chamber measuring 20 cm × 40.5 cm × 22 cm (L × W × H). Dividing walls are clear with small semicircular openings (3.5 cm radius) allowing access into each chamber. The middle chamber is empty, and the two outer chambers contain small, round wire cages (Galaxy Cup, Spectrum Diversified Designs, Inc., Streetsboro, OH) during testing. The mice were habituated to the entire apparatus with the round wire cages removed for 5 min. Mice were familiarized with a stranger mouse (B6 of the same sex being tested, habituated to the wire cage) in one of the wire cages in an outer compartment and another identical wire cage in the opposite compartment for 5 min, followed by removal for 5 min before initiating the test. For the assay, mice were returned to the middle chamber, this time with the original familiar mouse in its chamber and a new unfamiliar mouse (novel mouse) in the previously empty wire cage. Time spent in each chamber was recorded for 5 min. Twelve mice were assessed per group. Statistical analysis All data are expressed as the mean±s.e.m. ( N as indicated in the figure legends). Statistical test used to determine significant differences between treatment groups are indicated in the figure legends. Variance within groups was assessed by calculation of s.d. and variance was similar between groups that were compared. For all in vivo experiments, the treatment groups were blinded to the investigator. Mice were randomized to treatment groups, to control of potential effects of cage mates and litter effects. Group sizes for particular experiments were based on potential levels of efficacy compared with known positive controls (for example, chlordiazepoxide or cocaine) and power analysis. Normal distribution was confirmed for all experimental groups. How to cite this article : Banerjee, S. et al. Pharmacological targeting of the mammalian clock regulates sleep architecture and emotional behaviour. Nat. Commun. 5:5759 doi: 10.1038/ncomms6759 (2014).